A quantitative telomeric chromatin isolation protocol identifies different telomeric states Telomere composition changes during tumourigenesis, aging and in telomere syndromes in a poorly defined manner. Here we develop a quantitative telomeric chromatin isolation protocol (QTIP) for human cells, in which chromatin is cross-linked, immunopurified and analysed by mass spectrometry. QTIP involves stable isotope labelling by amino acids in cell culture (SILAC) to compare and identify quantitative differences in telomere protein composition of cells from various states. With QTIP, we specifically enrich telomeric DNA and all shelterin components. We validate the method characterizing changes at dysfunctional telomeres, and identify and validate known, as well as novel telomere-associated polypeptides including all THO subunits, SMCHD1 and LRIF1. We apply QTIP to long and short telomeres and detect increased density of SMCHD1 and LRIF1 and increased association of the shelterins TRF1, TIN2, TPP1 and POT1 with long telomeres. Our results validate QTIP to study telomeric states during normal development and in disease. Telomeres have crucial roles as guardians of the genome and tumour suppressors [1] . Telomere length shortens in the absence of telomerase due to the end replication problem and nucleolytic trimming of chromosome ends. Upon reaching a critically short size, telomeres trigger cellular senescence. Therefore, the absence of telomerase in most normal human somatic cells limits cellular lifespan and should suppress the growth of premalignant lesions that have lost normal cell cycle control [2] . On the other hand, telomerase is expressed during early embryogenesis and in some stem cells. This is important as deficiencies in telomerase genes lead to premature telomere shortening giving rise to degenerative syndromes with overlapping clinical features [3] . Telomere syndromes comprise dyskeratosis congenita, idiopathic pulmonary fibrosis, aplastic anaemia, Coats plus and others. Telomere function relies on its constituents, which includes telomeric DNA, telomeric proteins and the telomeric RNA TERRA [4] , [5] . Telomeric DNA consists of simple repetitive DNA sequences (5′-TTAGGG-3′/5′-CCCTAA-3′ repeats in humans) of several kilobases and terminates with single-stranded (ss) 3′ overhangs measuring a few hundred nucleotides [6] . Telomeric DNA is assembled with specialized telomere-binding proteins. The shelterin proteins include six abundant telomere-associated proteins [1] . The shelterin components TRF1 and TRF2 both bind directly to the double-stranded portion of telomeric DNA as homodimers [7] . POT1 binds the telomeric 3′ overhang [8] . TIN2, TPP1 and RAP1 associate with telomeres through protein interactions with TRF1, TRF2 and POT1. In senescent cells, short telomeres activate both ATM and ATR [9] . This telomeric state can be mimicked by experimental depletion of TRF2 from telomeres, which leads to the activation of ATM and depletion of POT1, which results in activation of ATR [10] . In addition to shelterin, an increasingly large number of less abundant and less-well characterized proteins were found in association with telomeres. These proteins also perform crucial functions, a fact that is underlined by the finding that they are mutated in several fatal degenerative syndromes. Some of them such as the Werner protein, Rtel1 and Pif1 are involved in the semiconservative DNA replication of telomeres for example to unwind G-quadruplex DNA structures, in which guanine bases of the telomeric G-strand associate through Hoogsteen hydrogen bonding to form tetrads [11] , [12] , [13] , [14] . Other important telomere factors are involved in the regulation of telomerase. The complete protein composition present at telomeres is not known nor are the changes in telomeric chromatin composition defined that occur during tumourigenesis, in short telomere syndromes and aging. Arguably one of the most important challenges of the telomere field is to define these changes and characterize their function. Here, we develop a quantitative telomeric chromatin isolation protocol (QTIP), which allows the comprehensive determination of telomere protein composition and the quantitative comparison of telomere protein compositions between cells that have different telomeric states. We implement QTIP to human cancer cells in which a telomeric DNA damage response is elicited by depletion of TRF2 or POT1, and to cancer cells with different telomere length, and we identify polypeptides that preferentially bind to long telomeres. The methodology developed here may also be adapted to other chromatin regions of the genome. Implementation of QTIP To compare telomeric chromatin composition from cells with different telomeric states, we developed QTIP. In QTIP, the proteins in the different cell populations to be compared are differentially labelled by incubating the cells in medium containing either heavy isotopes ([ 13 C 6 15 N 4 ]Arg (R10) and [ 13 C 6 15 N 2 ]Lys (K8)) or light isotopes (Arg (R0) and Lys (K0)) (Approach A, Fig. 1a ). Cells are mixed in a 1:1 ratio, chromatin is cross-linked with formaldehyde and sonicated upon cell lysis to obtain chromatin particles with DNA fragments of an average size of 200 bp (Approach A, Fig. 1a ). Telomeric chromatin is purified from the chromatin fraction by immunoprecipitation using affinity-purified polyclonal rabbit antibodies that were raised against full-length recombinant TRF1 and TRF2 and were covalently cross-linked to Protein G Sepharose beads. Independent batches of self-raised antibodies and also commercial antibodies were tested and found suitable for telomeric chromatin purification ( Supplementary Fig. S1 ). After extensive washing, purified material is eluted, the cross-links are reversed and proteins are fractionated by SDS–PAGE, trypsin digested and analysed by liquid chromatography–mass spectrometry (LC-MS/MS). The control experiment with unspecific immunoglobulin G (IgG) can be performed either in parallel on the same mixed cell population (Approach A, Fig. 1a ) or a separate immunoprecipitation can be performed on cells grown in a third stable isotope labelling by amino acids in cell culture (SILAC) medium (Approach B, Fig. 1a ). Thus in approach B, a triple SILAC strategy is employed which allows quantitative comparison of IgG contaminants by LC-MS/MS. This is optimal for the identification of new telomere interacting factors and their distinction from potential contaminants [15] . Approach A, on the other hand, minimizes experimental variations between the two samples and is suitable to compare variations of protein levels at telomeres between two different conditions. 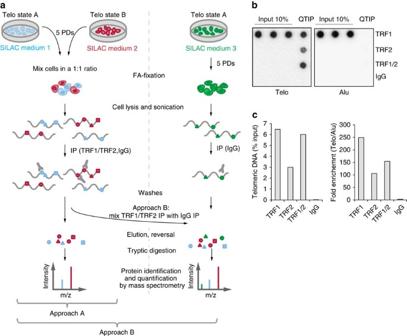Figure 1: Quantitative telomeric chromatin isolation protocol. (a) Workflow of QTIP. Approach A: Cells derived from telomeric state A (Telo state A) and telomeric state B (Telo state B) are cultivated in either light or heavy SILAC medium for five population doublings and then mixed in a 1:1 ratio, cross-linked with formaldehyde, lysed and sonicated. Telomeric chromatin is immunoprecipitated with affinity-purified antibodies against TRF1 and/or TRF2 or with a nonspecific control antibody (IgG). The enriched protein–DNA complexes are washed and eluted. Following the cross-link reversal, the proteins are subjected to tryptic digestion and identified and quantified by mass spectrometry. Peptides derived from the two conditions are distinguishable due to their mass differences. In Approach B, the immunoprecipitation with the nonspecific control antibody (IgG) is performed separately with control cells (Telo state A) using a third SILAC medium. Before elution, the immunoprecipitated complexes of the TRF1/TRF2 and the IgG IPs are mixed. The following steps are as in approach A (b) QTIP specifically enriches for telomeric DNA. Dot blot of DNA enriched by QTIP probed with a telomere-specific probe (Telo) or a probe against Alu-repeat DNA (Alu). (c) Quantification of the dot blot represented in (b). Representative result from one QTIP experiment. Figure 1: Quantitative telomeric chromatin isolation protocol. ( a ) Workflow of QTIP. Approach A: Cells derived from telomeric state A (Telo state A) and telomeric state B (Telo state B) are cultivated in either light or heavy SILAC medium for five population doublings and then mixed in a 1:1 ratio, cross-linked with formaldehyde, lysed and sonicated. Telomeric chromatin is immunoprecipitated with affinity-purified antibodies against TRF1 and/or TRF2 or with a nonspecific control antibody (IgG). The enriched protein–DNA complexes are washed and eluted. Following the cross-link reversal, the proteins are subjected to tryptic digestion and identified and quantified by mass spectrometry. Peptides derived from the two conditions are distinguishable due to their mass differences. In Approach B, the immunoprecipitation with the nonspecific control antibody (IgG) is performed separately with control cells (Telo state A) using a third SILAC medium. Before elution, the immunoprecipitated complexes of the TRF1/TRF2 and the IgG IPs are mixed. The following steps are as in approach A ( b ) QTIP specifically enriches for telomeric DNA. Dot blot of DNA enriched by QTIP probed with a telomere-specific probe (Telo) or a probe against Alu-repeat DNA (Alu). ( c ) Quantification of the dot blot represented in ( b ). Representative result from one QTIP experiment. Full size image We first determined which telomeric proteins are identified by QTIP in HeLa cells. The yield of telomeric DNA in QTIP samples was quantified by dot blot hybridization with a 32 P-labelled telomeric probe and compared with the signal with a probe against Alu-repeat DNA ( Fig. 1b,c ). Typically, 3–20% of telomeric DNA was recovered with a several hundred-fold enrichment over Alu-repeat DNA. QTIP using negative control IgG antibody did not give a detectable telomeric DNA signal ( Fig. 1b,c ). In QTIP purifications with antibodies against TRF1, TRF2 or a mixture thereof, we consistently identified peptides corresponding to all six shelterin components ( Table 1 ). None of the shelterin components was identified with negative control IgG. In addition, we identified peptides from several other reported telomere-associated components and factors known to assemble with telomere-associated components ( Supplementary Table S1 ). This includes the telomere end processing enzymes Apollo, Mre11, Nbs1 and Rad50; ORC complex components, DNA polymerase δ, the WRN interacting protein WRNIP1, which is required for efficient telomere replication [13] ; PNUTS [16] and subunits of the PNUTS containing PTW/PP1 phosphatase complex, which had not been previously characterized at telomeres [17] . Table 1 QTIP specifically enriches for all shelterin subunits. 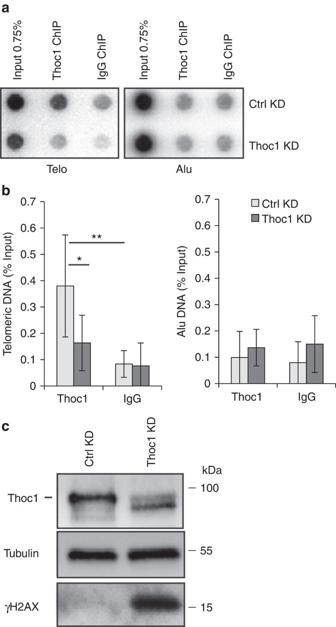Figure 2: QTIP identifies novel telomeric proteins. (a) Validation of Thoc1 as a novel telomeric protein. ChIP against endogenous Thoc1 in HeLa cells with short telomeres. Thoc1 ChIP in HeLa cells upon shRNA-mediated Thoc1 knockdown was performed as a specificity control for the antibody. ChIPed DNA was probed with a telomere-specific probe (Telo) and a probe against Alu-repeat DNA (Alu). (b) Quantification of Thoc1 ChIP as shown in (b). Error bars correspond to s.d. of results of four independent experiments (Student’st-test, *Pvalue <0.05, **Pvalue <0.005). (c) Western blot confirming knockdown of Thoc1 protein and increase of γH2AX phosphorylation upon Thoc1 knockdown. Full size table Identification of the THO complex at telomeres In addition to the factors listed in Table 1 and Supplementary Table S1 , we identified peptides from seven of the eight subunits of the THO and TREX complexes, LRIF1 and SMCHD1 (described below) at telomeres ( Table 2 ). THO has roles in mRNP biogenesis, connecting transcription elongation with RNA maturation and nuclear export, and preventing genetic instability [18] . Its function in the regulation of the long noncoding RNA TERRA at telomeres and telomere stability in Saccharomyces cerevisiae is characterized in a separate paper [19] . We validated the presence of the human Thoc1 subunit at telomeres in chromatin immunoprecipitation (ChIP) experiments with an antibody ( Fig. 2a,b ). Dot blot hybridization demonstrated specific enrichment of telomeric DNA over Alu-repeat DNA, when compared with negative control IgG. To control for specificity of the anti-Thoc1 antibody, we depleted Thoc1 by small hairpin RNA (shRNA) and observed reduced Thoc1 levels on western blots ( Fig. 2c ). Thoc1 depletion also led to an increase in γ-H2AX as expected, which is a marker for damaged DNA that accumulates in Thoc1-depleted cells [20] . Importantly, Thoc1 depletion also led to a significant reduction of the telomeric DNA signal in the ChIP experiments confirming the significance of the results ( Fig. 2b ). Additional polypeptides that were identified by QTIP but that are not yet validated as genuine telomere components by independent experiments can be accessed online ( Supplementary Data 1 ). Table 2 List of novel telomeric proteins identified by QTIP. Full size table Figure 2: QTIP identifies novel telomeric proteins. ( a ) Validation of Thoc1 as a novel telomeric protein. ChIP against endogenous Thoc1 in HeLa cells with short telomeres. Thoc1 ChIP in HeLa cells upon shRNA-mediated Thoc1 knockdown was performed as a specificity control for the antibody. ChIPed DNA was probed with a telomere-specific probe (Telo) and a probe against Alu-repeat DNA (Alu). ( b ) Quantification of Thoc1 ChIP as shown in ( b ). Error bars correspond to s.d. of results of four independent experiments (Student’s t -test, * P value <0.05, ** P value <0.005). ( c ) Western blot confirming knockdown of Thoc1 protein and increase of γH2AX phosphorylation upon Thoc1 knockdown. Full size image QTIP reveals protein changes at dysfunctional telomeres As mentioned in the introduction, both depletion of the double-stranded telomeric DNA binding factor TRF2 and the ss DNA binding factor POT1 induce dysfunctional telomeres, activating ATM and ATR signalling, respectively [10] . We established HeLa cell lines from which TRF2 or POT1 can be depleted by doxycycline (dox)-inducible expression of shRNAs from lentiviral vectors [21] ( Fig. 3a ). In this system, expression of a fusion protein of the strong repressor protein domain KRAB and the tetracycline repressor (tTR), which binds on either side of the H1 promoter to tetO sequences, represses transcription of the shRNA in the absence of dox. Repression is relieved upon addition of dox to the medium, which induces a conformational change in tTR-KRAB preventing its binding to tetO. We transduced HeLa cells consecutively with the repressor construct and shRNA constructs. After clonal selection using fluorescence-activated cell sorting (FACS) of dox-regulatable green fluorescent protein (GFP) expression, TRF2 knockdown was characterized in several clones. Western blot analysis of two clones showed efficient TRF2 depletion upon addition of dox, concomitant with an upregulation of the phosphorylated form of H2AX (γ-H2AX) indicating a DNA damage response ( Fig. 3b ). Furthermore, analysis of metaphase chromosome spreads of cells induced for 5 to 7 days showed that the TRF2 knockdown induced telomere fusions as expected for a functional depletion of this protein [22] ( Fig. 3d ). We also verified the amount of telomeric DNA in cells with dysfunctional telomeres, which did not vary significantly upon depletion of TRF2 ( Supplementary Fig. S2 ). POT1 reduction was assessed by qRT–PCR comparing messenger RNA levels in uninduced and induced cells ( Fig. 3c ). To confirm that the POT1 knockdown was activating DNA damage signalling specifically at telomeres, we performed ChIP with anti γ-H2AX antibodies that showed enrichment of telomeric DNA but not Alu-repeat DNA upon dox induction ( Fig. 3e ). Thus, the characterized HeLa cell lines allow regulatable telomere deprotection. 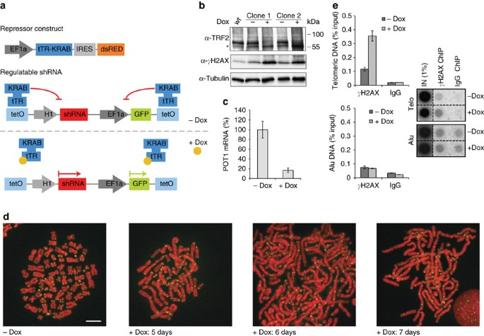Figure 3: Inducible TRF2 and POT1 knockdown generates dysfunctional telomeres. (a) Lentiviral vector-based strategy allowing dox-regulatable expression of shRNAs using tTR-KRAB repressor. (b–e) Characterization of HeLa cells upon induction of TRF2 or POT1 knockdown. (b) Western blot analysis revealing TRF2 depletion and H2AX phosphorylation after 4 days of dox induction. Asterisk: unspecific signal (two clones analysed). (c) POT1 messenger RNA depletion analysis by qPCR after 4 days of induction. Error bars correspond to s.d. of three independent experiments. (d) Metaphase chromosome spreads showing dramatic telomere fusions in cells induced for TRF2 depletion (scale bar, 6 μm). (e) γH2AX ChIP showing telomere-specific DNA damage signalling upon dox induction. Representative dot blot analysis is shown; s.d. are indicated. Average values are derived from three independent clones. Figure 3: Inducible TRF2 and POT1 knockdown generates dysfunctional telomeres. ( a ) Lentiviral vector-based strategy allowing dox-regulatable expression of shRNAs using tTR-KRAB repressor. ( b – e ) Characterization of HeLa cells upon induction of TRF2 or POT1 knockdown. ( b ) Western blot analysis revealing TRF2 depletion and H2AX phosphorylation after 4 days of dox induction. Asterisk: unspecific signal (two clones analysed). ( c ) POT1 messenger RNA depletion analysis by qPCR after 4 days of induction. Error bars correspond to s.d. of three independent experiments. ( d ) Metaphase chromosome spreads showing dramatic telomere fusions in cells induced for TRF2 depletion (scale bar, 6 μm). ( e ) γH2AX ChIP showing telomere-specific DNA damage signalling upon dox induction. Representative dot blot analysis is shown; s.d. are indicated. Average values are derived from three independent clones. Full size image We applied QTIP to one of the HeLa cell clones in which we could deplete TRF2 upon addition of dox. Cells were grown for five generations in medium containing heavy isotopes ([ 13 C 6 15 N 4 ]Arg (R10) and [ 13 C 6 15 N 2 ]Lys (K8)). Dox was added (+dox) during the last 4 days of cultivation with heavy isotopes to induce shRNA expression. These cells were then mixed with equal number of uninduced (−dox) cells grown for five doublings in medium containing medium isotopes ([ 13 C 6 ]]Arg (R6) and [4,4,5,5-D4]Lys (K4)) and processed ( Fig. 1a ). As TRF2 had been depleted in the +dox cells, we only used anti-TRF1 antibodies for QTIP. In parallel, an equal number of cells was grown in light SILAC medium (Arg (R0) and Lys (K0)) and subjected to immunoprecipitation with unspecific rabbit IgG. Before elution, the washed beads of the TRF1 and IgG immunoprecipitates were mixed ( Fig. 1a , Approach B). Comparing the ratio heavy/medium revealed changes at telomeres that occurred upon TRF2 depletion ( Fig. 4a ). As expected, TRF2 strongly decreased at telomeres from +dox cells ( Fig. 4a ). Interestingly, the shelterin components TRF1, TIN2, TPP1 and POT1 were also clearly reduced in TRF2-depleted cells suggesting that their association with telomeres is promoted by TRF2. RAP1 was also detected at telomeres; however, the low abundance of detected peptides did not allow quantification. When including the TRF1/IgG immunoprecipitation ratio performed in the scatter plot ( Fig. 4b ), we observed specific enrichment of telomeric proteins with the TRF1 antibody compared with the IgG control ( Fig. 4b ). This result underlines the suitability of the triple SILAC approach to distinguish telomeric proteins. The reproducibility of the technique was very good as assessed by comparing two independent QTIP experiments ( Supplementary Fig. S3 ). In addition to the discussed shelterins, several new candidate proteins showed increasing or decreasing levels at telomeres upon TRF2 depletion. Their putative association and biological function at telomeres will require validation and further characterization. 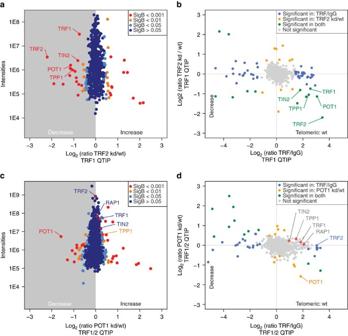Figure 4: QTIP reveals quantitative changes in protein composition at dysfunctional telomeres. (a) Scatter plot representing the log2ratio of a QTIP experiment with cells depleted for TRF2 versus uninduced control cells (wild type, wt). The significances of variations are indicated (top right). (b) Comparison of log2ratio (TRF2 kd/wt) to log2ratio of TRF1 versus IgG immunoprecipitation in wt. Proteins present at telomeres in wt condition and decreasing upon TRF2 kd are located in the bottom right panel. (c,d) Same as (a,b) but applied to POT1 knockdown. Figure 4: QTIP reveals quantitative changes in protein composition at dysfunctional telomeres. ( a ) Scatter plot representing the log 2 ratio of a QTIP experiment with cells depleted for TRF2 versus uninduced control cells (wild type, wt). The significances of variations are indicated (top right). ( b ) Comparison of log 2 ratio (TRF2 kd/wt) to log 2 ratio of TRF1 versus IgG immunoprecipitation in wt. Proteins present at telomeres in wt condition and decreasing upon TRF2 kd are located in the bottom right panel. ( c , d ) Same as ( a , b ) but applied to POT1 knockdown. Full size image QTIP analysis was also applied to the POT1-depleted HeLa cell clones using TRF1 and TRF2 antibodies. POT1-depleted (+dox) cells were grown with heavy isotopes, non-depleted (−dox) cells with medium isotopes and the IgG control was applied to cells grown with light isotopes. The scatter plot ( Fig. 4c ) revealed a strong depletion of POT1 at telomeres from +dox cells as expected. In contrast to the TRF2 knockdown, POT1 depletion was not accompanied by a concomitant decrease of the other five shelterin components. The specific decrease of POT1 was confirmed when integrating the IgG immunoprecipitation data in the scatter plot ( Fig. 4d , Supplementary Fig. S4 ). This result confirms that QTIP allows precise and quantitative analysis of changes in protein composition at telomeres. Increased association of proteins with long telomeres Having validated QTIP for the identification of changes in protein composition at telomeres, we compared by QTIP telomeres of different lengths. To induce telomere elongation, we stably transduced HeLa cells with constructs for the catalytic core components of telomerase hTERT and human telomerase RNA as described [23] and expanded the cells for ~35 population doublings. Telomere length analysis by Southern blotting ( Fig. 5a ) revealed an average telomere length of ~10 kb in parental HeLa cells (termed ‘short’) and an average telomere length of 30 kb in telomerase-transduced HeLa cells (termed ‘long’). The proteins in the two different HeLa cell populations were differentially labelled for five generations incubating the cells in medium containing either heavy isotopes ([ 13 C 6 15 N 4 ]Arg (R10) and [ 13 C 6 15 N 2 ]Lys (K8)) or light isotopes (Arg (R0) and Lys (K0)) ( Fig. 1a , Approach A). In consecutive experiments, the labelling with heavy and light amino acids was inverted for HeLa cells with long and short telomeres giving similar results ( Fig. 5b ). QTIP was performed with a mixture of anti-TRF1 and anti-TRF2 antibodies ( Fig. 5b ). Using QTIP, we recovered increased amounts of the shelterin components TRF1, TIN2, TPP1 and POT1 from HeLa cells with long telomeres ( Fig. 5b ). The increased association of POT1 and TPP1 with long telomeres is not due to a longer ss telomeric 3′ overhang, which is similar in the two cell lines ( Supplementary Fig. S5 ). TRF2 and RAP1 on the other hand were equally abundant at long and short telomeres. In addition, we observed a very strong increase of SMCHD1 (structural maintenance of chromosomes flexible hinge domain-containing protein 1) and LRIF1 (ligand-dependent nuclear receptor-interacting factor 1) at long telomeres ( Fig. 5b ). When performing QTIP in separate experiments with either anti-TRF1 or anti-TRF2 antibodies only, we also observed increased amounts of LRIF1 and SMCHD1 with long telomeres ( Fig. 5c,d ). LRIF1 is a nuclear protein identified in a 2-hybrid screen with RARα. LRIF1 also interacts with histone deacetylases [24] repressing reporter gene expression. SMCHD1 localizes to the inactive X chromosome in females and has a role in the maintenance of X inactivation and hypermethylation of CpG islands [25] . Interestingly, LRIF1 (also referred to as HBiX1) and SMCHD1 were recently shown to physically interact and to be important for compacting H3K9me3-rich and XIST-H3K27me3 domains at the inactive X chromosome in human cells [26] . 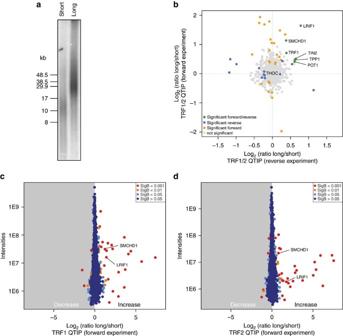Figure 5: Identification of quantitative differences between telomeric proteins at short and long telomeres by QTIP. (a) Telomere restriction analysis of isogenic Hela cells with short or long telomeres used for QTIP experiments. (b) Scatter plot representing the log2(ratio long/short) from two independent biological TRF1/2 QTIP experiments. Proteins significantly changing between short and long telomeres in both experiments are indicated by a green dot, whereas factors that are not changing are represented by a grey dot (for example, THO complex subunits). (c) Intensities versus log2(ratio long/short) of a TRF1 QTIP experiment are depicted. (d) Intensities versus log2(ratio long/short) of a TRF2 QTIP experiment are depicted. Figure 5: Identification of quantitative differences between telomeric proteins at short and long telomeres by QTIP. ( a ) Telomere restriction analysis of isogenic Hela cells with short or long telomeres used for QTIP experiments. ( b ) Scatter plot representing the log 2 (ratio long/short) from two independent biological TRF1/2 QTIP experiments. Proteins significantly changing between short and long telomeres in both experiments are indicated by a green dot, whereas factors that are not changing are represented by a grey dot (for example, THO complex subunits). ( c ) Intensities versus log 2 (ratio long/short) of a TRF1 QTIP experiment are depicted. ( d ) Intensities versus log 2 (ratio long/short) of a TRF2 QTIP experiment are depicted. Full size image To validate the identified changes in telomeric chromatin composition upon telomere elongation, we performed with the same HeLa cells additional ChIP experiments using antibodies against selected telomere components and quantified telomeric DNA and Alu-repeat DNA as a negative control in the ChIP samples ( Fig. 6 ). For TRF1, we confirmed in ChIP experiments that higher absolute amounts of TRF1 are present at telomeres when they are long but that the relative association, reflecting the density of binding is slightly reduced. Alternatively, long telomeres may contain longer stretches devoid of TRF1 ( Fig. 6a , Supplementary Fig. S6 ). For TRF2, ChIP experiments indicated an even stronger density decrease at long telomeres than for TRF1, explaining why no difference in absolute TRF2 quantity was detected by QTIP between long and short telomeres. This, therefore, indicates that TRF2 density at long telomeres is lower or that long telomeres contain larger stretches of telomeric DNA lacking TRF2 ( Fig. 6a , Supplementary Fig. S6 ). MRN complex (Mre11/Rad50/Nbs1) association with functional telomeres is mediated by TRF2 (ref. 27 ). Therefore, one would expect similar results for TRF2 and Mre11 in QTIP and ChIP experiments when comparing short and long telomeres. Indeed, as for TRF2, we did not recover more Mre11 from cells with long telomeres. Mre11 also showed the same trend as TRF2 in the ChIP experiment, associating with lower relative amounts of telomeric DNA at long telomeres ( Fig. 6b , Supplementary Fig. S6 ). 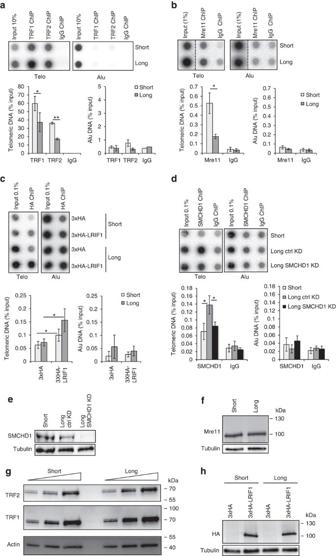Figure 6: Validation of variations identified by QTIP of short and long telomeres. (a–d) ChIP experiments against the indicated proteins performed in isogenic HeLa cell lines with either short or long telomeres. Error bars correspond to s.d. of three independent experiments (Student’st-test, *Pvalue <0.05, **Pvalue <0.005). (e–h) Western blots showing no variation in total protein levels between HeLa cells with short and long telomeres of the proteins used for ChIP in (a–d). Anti-SMCHD1 antibody validation for immunoblotting is shown inSupplementary Fig. S8. Figure 6: Validation of variations identified by QTIP of short and long telomeres. ( a – d ) ChIP experiments against the indicated proteins performed in isogenic HeLa cell lines with either short or long telomeres. Error bars correspond to s.d. of three independent experiments (Student’s t -test, * P value <0.05, ** P value <0.005). ( e – h ) Western blots showing no variation in total protein levels between HeLa cells with short and long telomeres of the proteins used for ChIP in ( a – d ). Anti-SMCHD1 antibody validation for immunoblotting is shown in Supplementary Fig. S8 . Full size image To study telomere association of LRIF1 by ChIP, we expressed 3xHA-tagged LRIF1 upon transient transfection in the HeLa cells with long and short telomeres and performed ChIP with anti-HA antibodies ( Fig. 6c ). The telomeric signal obtained with cells expressing 3xHA-LRIF1 was significantly higher than in cells expressing the empty vector control (3xHA). Strikingly, the immunopurification yielded higher levels of telomeric DNA from long telomeres not only in absolute but also relative amounts. This result is consistent with the QTIP analysis ( Fig. 5 ) supporting the notion that LRIF1 preferentially binds to long telomeres ( Fig. 6c , Supplementary Fig. S6 ). For SMCHD1, we performed ChIP using antibodies against the endogenous protein ( Fig. 6d ). Telomeric DNA was specifically enriched when compared with the signal obtained with nonspecific control antibodies (IgG). Furthermore, small interfering RNA (siRNA)-mediated depletion of SMCHD1 ( Fig. 6e ) led to a decrease of the telomeric signal, indicating specificity of the antibody for SMCHD1. As seen for LRIF1, immunopurification of SMCHD1 yielded more telomeric DNA in absolute and relative amounts from long telomeres confirming the conclusion from the QTIP experiment that SMCHD1 preferentially associates with long telomeres ( Fig. 6d , Supplementary Fig. S6 ). We tested on western blots of whole cell lysates, whether telomere length had an impact on protein abundance of the factors under investigation ( Fig. 6f–h ). However, TRF1, TRF2, Mre11, SMCHD1 and 3xHA-LRIF1 levels did not change significantly upon telomere elongation. Therefore, the differences seen in telomere association with long and short telomeres are not due to changes in protein abundance. One of the biggest challenges in the telomere field is to identify the molecular changes at telomeres that occur in cancer and in telomere syndromes. With QTIP, we develop here a method that allows purification of telomeric chromatin and its analysis by mass spectrometry. We apply QTIP to cells with different telomeric states, including dysfunctional telomeres or telomeres with various lengths, and we demonstrate that QTIP is suitable to identify quantitative differences between diverse telomeric states. A method termed PICh in which telomeres are partially denatured and affinity purified via antisense hybridization techniques was described before [28] . In both, QTIP and PICh, telomeric chromatin is cross-linked in vivo and subsequently purified. Therefore, both methods represent a significant advance over attempts to study telomeric chromatin upon reconstitution in vitro . However, QTIP and PICh have the following significant differences. PICh includes an RNase step, which may lead to the loss of TERRA-dependent telomeric factors. This may explain why PICh did not identify subunits of the THO/TREX complexes except THOC4. Additionally, PICh requires 60 × higher cell numbers than QTIP. Most significantly, QTIP uses the SILAC methodology and allows quantitative comparison of telomeric states of different cells. Both methods identified all shelterin components but for telomere-associated proteins, there is only a partial overlap ( Supplementary Data 1 and Supplementary Fig. S7 ). Thus, both methods provide complementary information. We identify by QTIP seven THO/TREX subunits at telomeres and we validate telomere association of Thoc1 by ChIP. The THO complex is involved in RNA maturation [18] and its presence at telomeres suggests roles in TERRA biogenesis. We were so far unable to confirm this notion for human TERRA but our laboratory has recently obtained data in S. cerevisiae, which demonstrate that telomere association of THO is conserved in yeast and that THO removes DNA–RNA hybrids from yeast telomeres [19] . The QTIP experiments performed with cells depleted for TRF2 or POT1 demonstrate that we can identify quantitative changes of the target telomeric protein and the effect of the knockdown on the protein complex partners. Additionally, we identified several new candidate telomere proteins, which were enriched in the TRF1/2-QTIP over the IgG control at wt telomeres and whose abundance changed at telomeres upon TRF2 or POT1 depletion. These proteins will require individual validation and characterization. We also discover using QTIP that LRIF1 and SMCHD1 preferentially associate with long telomeres. These results were confirmed in ChIP experiments, which further indicated an increased density for both of these factors at long telomeres. SMCHD1 is also associated with the inactive X chromosome sustaining methylation of CpG island [25] and X chromosome compaction [26] . A similar function at telomeres might contribute to the preferential silencing of CpG island containing TERRA promoters at long telomeres [29] , [30] . As LRIF1 has been reported to interact with histone deacetylases [24] , it might also reinforce the heterochromatic nature of long telomeres. A role in telomeric heterochromatin is also consistent with the recent observation of its interaction with SMCHD1 (ref. 26 ). We also identify using QTIP differences for shelterin components at long and short telomeres. With long telomeres, we recovered more TRF1, TIN2, TPP1 and POT1 by QTIP. For TRF1, we confirmed in ChIP experiments that higher absolute amounts of TRF1 are present at telomeres when they are long but that the relative association and therefore the density of binding is reduced. Alternatively, long telomeres may contain longer stretches that lack TRF1. For TRF2, the ChIP experiments indicated that the difference in density at long telomeres drops more substantially than for TRF1 explaining why no difference was detected for TRF2 by QTIP between long and short telomeres. Our results therefore reinforce the notion that shelterin may exist at telomeres not only as a six-subunit complex but that shelterin sub-complexes of various composition may associate with chromosome ends. Shelterin sub-complexes have been seen in previous studies in nuclear extracts [31] , [32] , [33] and absolute quantifications of shelterin components in cells demonstrated that they are not stoichiometric [34] . Future work will try to elucidate the function of SMCHD1 and LRIF1 at long telomeres and validate telomere association of other identified candidates. We anticipate that QTIP may find broad and useful applications for the diagnosis and characterization of cancer types, telomere syndromes and for addressing how telomeric chromatin composition may change during development. More generally, our approach might be applicable to other chromatin-interacting complexes such as chromatin modifiers or transcription factors to study composition and modular changes of a variety of chromatin-associated complexes. Cell culture and transfections HeLa super-telomerase and HeLa control cells were generated by transducing HeLa cells (ATCC) with retroviruses expressing hTERT from the LTR (long terminal repeat) promoter and human telomerase RNA from the U1 promoter or with empty vectors, respectively [23] . For Thoc1 shRNA knockdown and LRIF1 expression, cells were transfected with Lipofectamine 2000 (Invitrogen). shRNA-transfected cells were selected with puromycin (1 μg ml −1 , InvivoGen) starting 24 h after transfection during 4 days. Thoc1 ChIP experiments were performed 5 days after transfection. LRIF1 ChIP experiments were performed 48 h after transfection. For SMCHD1 siRNA KD, cells were transfected with INTERFERin (Polyplus) and with siRNA against SMCHD1 (Hs_KIAA0650_3, Qiagen) or a negative control siRNA (AllStars Negative Control siRNA, Qiagen). SMCHD1 ChIP experiments were performed 48 h post transfection. The inducible cell lines were generated by infection of HeLa cells with second-generation lentiviral vectors containing the tTR-KRAB construct and dsRED marker. Subsequently, cells were infected with the second lentiviral vector containing the H1 promoter-controlled shRNA sequence and GFP marker. FACS allowed selection of single cells and establishment of clonal populations. Inducible cell lines were grown in Dulbecco's Modified Eagle Medium (DMEM) supplemented with 10% Tet System Approved FBS (Clontech), 100 U ml −1 penicillin and 100 μg ml −1 streptomycin (Gibco). Dox was used at 1 μg ml −1 for induction. SILAC labelling was performed by cultivating cells for five population doublings in SILAC DMEM supplemented with 10% dialysed FCS, 100 U ml −1 penicillin and 100 μg ml −1 streptomycin (Gibco), 25 mg l −1 arginine (light arg: 12 C/ 14 N, medium arg: 13 C or heavy arg: 13 C/ 15 N), 46 mg l −1 lysine (light lys: 12 C/ 14 N, medium lys: D or heavy lys: 13 C/ 15 N) and 200 mg l −1 Proline. SILAC reagents were from the Thermo Fisher Scientific group with the exception of heavy and medium arginine and lysine (Cambridge Isotopes Laboratories). In the forward experiment, HeLa control cells were labelled with light amino-acid sets. In the reverse experiment, they were labelled with heavy amino acids. Lentiviral vectors production and cell transduction Lentiviral vectors were produced [21] . Plasmids pMD2G (55 μg), pCMVR8.74 (102 μg) and pLV-tTR-KRAB-red or pLV-T derivatives, to express shRNA sequences (157 μg) (kind gifts from Didier Trono), were mixed for co-transfection of HEK293T cells on 7 × 150 mm dishes using the calcium phosphate method (CalPhos Mammalian Transfection Kit, Clontech). Cells were incubated overnight and the supernatant was replaced by fresh DMEM medium containing 10% FCS. Supernatant was collected after 8 h and replaced by fresh medium for another 12 h. The harvested supernatant was cleared using a 0.22 μm filter unit (Stericup, Millipore) before concentration by ultracentrifugation for 2 h at 50,000 g, 16 °C (Beckman Coulter: Ultra-Clear tubes No. 344058, Rotor SW32Ti). The pellets were resuspended in a minimal volume of cold phosphate-buffered saline (PBS) and the lentiviral particles frozen at −80 °C. HCT116 cells were used for determination of lentiviral vector titre by FACS analysis of GFP or dsRED fluorescence performed 3 days post transduction. Subsequently, HeLa cells were infected with highly concentrated lentivirus using increasing multiplicities of infection ranging from 1–100. Expression of recombinant TRF1 and TRF2 Recombinant 6xHis-S-TRF1 and 6xHis-S-TRF2 were expressed in Rosetta DE3 pLysS competent cells (Novagen, 70956-4) from a pET-30a(+) plasmid (kind gifts from Daniela Rhodes). The recombinant proteins were purified on Ni-NTA agarose (Qiagen), dialysed against 1 × PBS, 10% glycerol (SnakeSkin Pleated Dialysis Tubing, 10 kDa, Thermo Fisher Scientific Group) and concentrated in an Amicon Ultra (30 kDa, Merck-Millipore). Antisera production against TRF1 and TRF2 Rabbits were immunized using four injections during an 87-day programme (Eurogentec). For each injection, 120 μg of native recombinant TRF1 or TRF2 were used. Antisera from final bleed were used for purification of the antibodies. Affinity purification of TRF1 and TRF2 sera Five milligrams of recombinant 6xHis-S-TRF1 or 6xHis-S-TRF2 protein (expressed in Rosetta DE3 pLysS competent cells (Novagen, 70956-4)) was bound to 1 ml Affigel-10 (TRF2) or Affigel-15 (TRF1) (Bio-Rad). Five millilitres of serum (TRF1 #605 448, TRF2 #605 782) was incubated with the Affigel matrix at 4 °C for 3 h. Unbound antibodies were drained and saved on ice. Bound antibodies were washed with 4 ml 2 × PBS and eluted 10 times with 1 ml 0.2 M glycine pH 2.5, 0.5 M NaCl. The eluted antibodies were immediately neutralized with saturated Tris base. The Affigel matrix was regenerated by washing with 2 ml 2 × PBS and the serum was loaded onto the matrix a second time. The following steps were performed as above. Antibody containing fractions were pooled, dialysed against 1 × PBS, 8.7% glycerol (SnakeSkin Pleated Dialysis Tubing, 10 kDa, Thermo Fisher Scientific Group) and concentrated in an Amicon Ultra (30 kDa, Merck-Millipore). Dimethyl Pimelimidate coupling of anti-TRF1 and anti-TRF2 to Protein G Sepharose Affinity-purified anti-TRF1 or anti-TRF2 were incubated for 1 h at room temperature with Protein G Sepharose 4 Fast Flow (GE Healthcare Life Sciences). The sepharose was washed once with 10 volumes 1 × PBS and twice with 10 volumes 0.2 M sodium borate pH 9.0. 20 mM dimethyl pimelimidate (DMP-solid, Sigma-Aldrich) was added to the sepharose resuspended in 10 volumes 0.2 M sodium borate pH 9.0. After 30 min at room temperature, the reaction was stopped by washing the sepharose twice with 10 volumes of 0.2 M ethanolamine pH 8.0. The sepharose was incubated for an additional 2 h in 10 volumes 0.2 M ethanolamine at room temperature, washed extensively with 1 × PBS and resuspended in 1 volume of ChIP dilution buffer. QTIP In approach A, equal amounts of HeLa control and HeLa super-telomerase cells grown in either light or heavy SILAC medium were mixed in a 1:1 ratio. Cells were washed twice in PBS and cross-linked in 1% formaldehyde-1 × PBS for 15 min at 30 °C. Glycine (pH 2.5) was added to 125 mM in order to quench the reaction before washing the cells twice with PBS. Cells were lysed in lysis buffer (1% SDS, 10 mM EDTA pH 8.0, 50 mM Tris pH 8.0, EDTA-free protease inhibitor complex (Roche)) and incubated for 5 min at room temperature, centrifuged for 5 min at 1,500 g, washed once in lysis buffer and centrifuged as above. The chromatin-enriched pellets were resuspended in lysis buffer and sonicated during 30 cycles with 30 s ON and 30 s OFF per cycle using a Bioruptor (Diagenode, Twin, High Energy setting) or 30 min using a Focused-Ultrasonicator (E220, Covaris, duty: 5.0, PIP: 140, cycles: 200, amplitude: 0, velocity: 0, dwell: 0, 12 × 12-mm glass tubes with AFA fibre) replacing SDS in lysis buffer by 0.1% Na-deoxycholate, 0.25% sodium lauroyl sarcosinate. The sonicated lysate was centrifuged at 4 °C for 15 min at 20,000 g. The supernatant was diluted in 2 volumes of ChIP dilution buffer (0.75% Triton X-100, 10 mM EDTA pH 8.0, 50 mM Tris-HCl pH 8.0, 600 mM NaCl) and precleared for 1 h at 8 °C with Protein G Sepharose 4 Fast Flow (GE Healthcare Life Sciences). The precleared lysate (corresponding to 1 × 10 8 mixed cells, 5 × 10 7 cells per condition) was incubated with either affinity-purified TRF1 (rabbit serum 448), TRF2 (rabbit serum 782), TRF1 and TRF2 or normal rabbit IgG (sc-2027, Santa Cruz Biotechnology), using 175–230 μg of combined TRF1/TRF2 antibody and normal rabbit IgG (optimal amount determined by titration for telomeric DNA recovery efficiency), covalently coupled to Protein G Sepharose 4 Fast Flow with DMP (Sigma-Aldrich). The ChIP was performed at 8 °C overnight. Beads were washed with wash buffer 1 (0.1% SDS, 1% Triton X-100, 2 mM EDTA pH 8.0, 20 mM Tris pH 8.0, 300 mM NaCl), wash buffer 2 (0.1% SDS, 1% Triton X-100, 2 mM EDTA pH 8.0, 20 mM Tris pH 8.0, 500 mM NaCl), wash buffer 3 (500 mM LiCl, 1% NP-40, 1% Na-deoxycholate, 1 mM EDTA, 10 mM Tris pH 8.0) and twice with wash buffer 4 (1 mM EDTA, 10 mM Tris pH 8.0). DNA–protein complexes were eluted with 2.5 bead volumes of 0.5 M NH 4 OH at 37 °C. The eluates were vacuum-dried in a speed vac, resuspended in Laemmli buffer, and cross-links were reversed for 25 min at 95 °C. The material was separated on a 10% Mini Protean TGX (Bio-Rad) and stained with Simply Blue Safe Stain (Invitrogen). In approach B, cells from conditions A and B were grown in heavy and medium SILAC medium and mixed in a 1:1 ratio for TRF1/TRF2 ChIP similarly to approach A. Control cells, grown in light SILAC medium were processed in parallel and used for rabbit normal IgG ChIP. After overnight incubations, beads were washed separately as described above and beads from TRF1/TRF2 ChIP and normal IgG were combined at the end of wash 4 for a common elution step as described for approach A. Plasmids The Thoc1 shRNA vector was generated by cloning the targeting double-stranded DNA oligonucleotides into pSUPER-Puro [35] digested with BglII and HindIII, using the following 19 nucleotides target sequence: 5′-GGAAGATAATGATGCTCTA-3′. The coding sequence of human LRIF1 was cloned from HeLa cDNA and inserted into a pCDNA6-3xHA vector backbone (Invitrogen) using the In-Fusion HD cloning kit (Clontech). A cassette containing an H1 promoter sequence and the TRF2 shRNA sequence 5′-GCGCATGACAATAAGCAGA-3′ or the POT1 shRNA sequence 5′-GCTATCTGCTACAATACTT-3′ were excised from shRNA vector construct described above and cloned into a pLV-T-derived vector using the EcoRI and SalI restriction sites. Telomere restriction fragment analysis and G-overhang analysis For telomere restriction fragment analysis and telomeric G-overhang analysis, genomic DNA was isolated using the Wizard Genomic DNA Purification Kit (Promega). RsaI and HinfI restriction-digested DNA was separated by pulse-field gel electrophoresis on 1% agarose in 0.5 × TBE at 5 V cm −1 for 16 h at 14 °C with switch times ramped from 0.5 to 6 s. Telomeric DNA was denatured and detected by in-gel hybridization [23] . For G-overhang analysis, genomic DNA was or was not treated with ExoI (40 U ExoI/4 μg DNA, overnight at 37 °C). Following phenol extraction and ethanol precipitation, genomic DNA was digested with RsaI and HinfI and resolved by pulse-field electrophoresis as described above for 14 h. For G-overhang analysis, the gel was dried (50 °C) and first hybridized under native conditions (50 °C) for detection of ss telomeric DNA, before denaturation and a second hybridization for total telomeric DNA. The 32 P-labelled telomeric DNA probe was prepared as for ChIP analysis (see below). For washes, the gel was rinsed in 4 × SSC and incubated for 30 min in 4 × SSC at room temperature, followed by successive 30 min washes at 50 °C in 4 × SSC/0.5% SDS and 2 × SSC/0.5% SDS. Metaphase spreads analysis Following dox induction, cells were harvested and processed for metaphase spreads and fluorescent in situ hybridization as previously described using a Cy3-OO-(CCCTAA) 3 probe and 4′,6-diamidino-2-phenylindole staining [4] . RNA isolation and qRT–PCR Total RNA was isolated using the NucleoSpin RNA II kit (Macherey-Nagel) including a DNase digestion step on the column. For reverse transcription, 1 μg RNA and random primers were used with SuperScript III Reverse Transcriptase according to instructions (Invitrogen, Life Technologies). For real-time PCR, we used the Power SYBR Green Mix (Applied Biosystems) and the Applied Biosystems 7900HT Real-Time PCR System following standard procedures. Oligonucleotides sequences were: 5′-TCAGTCTGTTAAACTTCATTGCCC-3′ (POT1, forward), 5′-TGCACCATCCTGAAAAATTATATCC-3′ (POT1, reverse), 5′-TCCCTGGAGAAGAGCTACGA-3′ (β-actin, forward), 5′-AGCACTGTGTTGGCGTACAG -3′ (β-actin, reverse). In-gel digestion and LC-MS/MS Entire lanes of SDS–PAGE gels were sliced into pieces. The gel pieces were first washed twice for 20 min in 50% ethanol, 50 mM ammonium bicarbonate (AB, Sigma-Aldrich) and dried down by vacuum centrifugation. Sample reduction was then performed with 10 mM dithioerythritol (DTE, Merck-Millipore) at 56 °C for 1 h. A washing–drying step was performed as described above before alkylation of samples with 55 mM iodoacetamide (IAA, Sigma-Aldrich) for 45 min at 37 °C protected from light. Samples were then washed and dried again before storing them on ice. Digestion was performed overnight at 37 °C using modified mass spectrometry grade trypsin (Trypsin Gold, Promega) at a concentration of 12.5 ng μl −1 in 50 mM AB and 10 mM CaCl 2 . Resulting peptides were extracted twice for 20 min in 70% ethanol, 5% formic acid (FA, Merck-Millipore) with permanent shaking. Finally, samples were dried down by vacuum centrifugation and stored at −20 °C until LC-MS/MS measurements. Extracted peptides were resuspended in 2% acetonitrile (ACN, Biosolve), 0.1% FA for LC-MS/MS injections. Nano flow separations were performed on a Dionex Ultimate 3000 RSLC nano UPLC system (Thermo Fisher Scientific) on line connected with an Orbitrap Elite Mass Spectrometer (Thermo Fisher Scientific) piloted with Xcalibur (version 2.1) and Tune (version 2.5.5). A home-made capillary precolumn (Magic AQ C18; 3 μm-200 Å; 2 cm × 100 μm ID) was used for sample trapping and cleaning. Analytical separation was then performed using a C18 capillary column (Nikkyo Technos; Magic AQ C18; 3 μm-100 Å; 15 cm × 75 μm ID) at 250 nl min −1 . Samples were separated over a 130-min biphasic gradient ranging from 1.98% ACN, 0.099% FA (aqueous) to 81% ACN, 0.09% FA (organic). Each sample was injected in duplicates and analysed using a data-dependent acquisition mode with a dynamic exclusion of 40 s. The thirty most intense parent ions from each MS survey scan (m/z 300–1,800) were selected for subsequent linear ion trap tandem mass spectrometry (MS/MS) fragmentations by CID (Collision Induced Dissociation). Orbitrap MS survey scans resolution was set at 60,000 (at 400 m/z) and fragments were measured at low resolution into the Linear Ion Trap. A threshold of 500 counts was applied to trigger the fragmentation and singly charged ions were excluded. Source and fragmentation parameters were set as follow: capillary voltage 1.9 kV; capillary temperature 240 °C; normalized collision energy, 35%; activation Q, 0.25; activation time, 10 ms. Assigning peptide sequences using Andromeda SILAC labelled data were analysed with MaxQuant version 1.2.2.5 and 1.3.0.5 against the UniProt human database release 2012_04 (86747 sequences). MaxQuant generates a concatenated decoy database complemented with common contaminant sequences to determine the false discovery rate and to exclude false positive hits. Mass spectra were searched with an initial mass tolerance of 7 p.p.m. in MS mode and 0.5 kDa in MS/MS mode. Up to two missed cleavages were allowed. Carbamidomethylation was set as a fixed modification, whereas oxidation (M) and acetylation (protein N-term) (and phosphorylation (STY) only in the approach B) were considered as variable modifications. The minimal peptide length was set to six amino acids (seven in MaxQuant 1.3.0.5) and at least two (unique+razor) peptides were required for protein identification. A cut-off was fixed at 1% DR at the peptide and protein level. Reverse and contaminant sequences were removed and proteins with a posterior error probability lower than 0.1 were accepted for further data treatment. Protein quantification was performed with razor and unique peptides, using only unmodified, oxidated (M) and acetylated (protein N-term) peptides. A minimum of two ratio counts was required to quantify proteins. Data analysis SILAC ratios determined using MaxQuant were further processed to assess the significance of outlier ratios using Perseus, the statistical tool integrated in the MaxQuant software suite [36] . For our data set, we report significant ratios based on significance B with a Benjamin–Hochberg corrected P value threshold of 0.05. Further statistical treatments and graphical displays were performed using home-made programs written in R ( http://www.r-project.org/ ). To facilitate the comparison of the relative merits of QTIP versus the previously established PICh [28] , the list of proteins identified using approach A ( Supplementary Data 1 ) was rank sorted in the same way as done by Déjardin and Kingston [28] with slight modifications. Briefly, the ratio between telomeric or unspecifically bound proteins was calculated by dividing the number of razor and unique peptides identified per protein in each telomeric immunoprecipitation (TRF1, TRF2, TRF1/2 IPs) by those identified in the control immunoprecipitation (IgG IPs). This reflects the enrichment in telomeric IP. In case of no identification in one or the other condition, the value 0 was replaced by 0.059 (ratio between the number of peptides of the protein of the list generating the largest number of razor and unique peptides to the total number of proteins identified within the whole sample). Proteins were sorted according to this calculated ratio from high to low. Only proteins with a ratio above 2 were considered. The list was finally ranked using the calculated ratio of number of peptides per protein to the protein size as done by Déjardin and Kingston [28] . Proteins with less than five unique/razor peptides were not considered. ChIP ChIP for Mre11, TRF1, TRF2, HA, SMCHD1 and γ-H2AX was performed by preparing a chromatin-enriched extract as in QTIP. The sonicated lysate was diluted with four volumes of IP dilution buffer (1.2 mM EDTA pH 8.0, 1.1% Triton X-100, 16.7 mM Tris pH 8.0, 300 mM NaCl) and incubated with the corresponding antibody: 2 μg anti-Thoc1 (GTX118740, Genetex), 3 μl Mre11 (NB100-142, Novus Biologicals), 20 μl rabbit anti-TRF1 serum 488, 20 μl of rabbit anti-TRF2 serum 782, 2.3 μg anti-HA (AB9110, Abcam), 4 μg anti-γ-H2AX (Millipore 05–636), 3 μg anti-SMCHD1 (A302-871A, Bethyl Laboratories), corresponding amount of normal rabbit or mouse IgG (sc-2027 or sc-2025, Santa Cruz Biotechnology) and 20 μl of Protein G Sepharose 4 Fast Flow at 4 °C overnight. Beads were washed as in the QTIP. Elution and cross-link reversal was performed at 65 °C overnight in 1% SDS, 0.1 M NaHCO 3 , 0.5 mM EDTA pH 8.0, 20 mM Tris pH 8.0, 10 μg DNase-free RNase (Roche). For DNA extraction, the QIAquick PCR Purification kit (Qiagen) was used. Telomeric and Alu-repeat DNA were detected successively [37] . Telomeric DNA was detected using a probe [4] that was generated as follows: a template mixture of 1–5 kb long telomeric DNA fragments was synthesized by ligating double-stranded telomeric DNA oligonucleotides ((TTAGGG) 5 , (CCCTAA) 5 ) that were amplified by PCR. The probe was random primer labelled with α- 32 P-dCTP and cold dTTP and dATP (for detection of the TTAGGG strand). Alu-repeat DNA was detected using a 5′ 32 P-labelled oligonucleotide probe (5′-GTGATCCGCCCGCCTCGGCCTCCCAAAGTG-3′) that was hybridized at 55 °C. ChIP with Thoc1 antibody was performed by preparing a chromatin-enriched extract as above. After the sonication step, 200 mM KCl was added to precipitate the SDS. After 5 min incubation on ice, the lysate was centrifuged at 4 °C for 15 min at 20,000 g. The supernatant was supplemented with 0.5% NP-40, 2 μg anti-Thoc1 (GTX118740, Genetex) or corresponding amount of normal rabbit IgG (sc-2027, Santa Cruz Biotechnology) and 20 μl of protein G sepharose 4 Fast Flow and incubated at 4 °C overnight. Beads were washed five times in RLN buffer (140 mM NaCl, 50 mM Tris pH 8, 1.5 mM MgCl 2 , 0.5% NP-40). The following steps were performed as described above. Immunoblots 0.5–1 × 10 5 cells were boiled for 5 min in Laemmli buffer and separated on a 4–20% Mini Protean TGX (Bio-Rad). Standard immunoblot protocols were used with the following antibodies: anti-Thoc1 (GTX118740, Genetex, diluted 1/1,000), anti-HA (AB9110, Abcam, diluted 1:1,000), anti-γ-H2AX (Millipore 05–636, diluted 1:1,000), anti-tubulin (T9026, Sigma-Aldrich, diluted 1:1,000), anti-Mre11 (NB100-142, Novus Biologicals, diluted 1/1,000), anti-TRF1 (T1948, Sigma-Aldrich, diluted 1:1,000), anti-TRF2 (05–521, Merck-Millipore, diluted 1:1,000) anti-SMCHD1 (A302-871A, Bethyl Laboratories, diluted 1/2,000), anti-actin (sc-1616, Santa Cruz Biotechnology, diluted 1/1,000). Secondary HRP-conjugated antibodies against rabbit (W4011, Promega, diluted 1:3,000), mouse (W4021, Promega, diluted 1:3,000) or goat (sc-2953, Santa Cruz Biotechnology, diluted 1:3,000) IgG were used to reveal the primary antibodies. Luminata Forte Western HRP Substrate (Merck-Millipore) was used for signal detection. Validation of the anti-SMCHD1 antibody is shown in Supplementary Fig. S8 . Accession codes: The mass spectrometry proteomics data have been deposited in ProteomeXchange ( http://proteomecentral.proteomexchange.org ) via the PRIDE partner repository [38] with the data set identifier PXD000243. How to cite this article: Grolimund, L. et al . A Quantitative Telomeric Chromatin Isolation Protocol identifies different telomeric states. Nat. Commun. 4:2848 doi: 10.1038/ncomms3848 (2013).